TNFR1 mediates TNF-α-induced tumour lymphangiogenesis and metastasis by modulating VEGF-C-VEGFR3 signalling Inflammation and lymphangiogenesis are two cohesively coupled processes that promote tumour growth and invasion. Here we report that TNF-α markedly promotes tumour lymphangiogenesis and lymphatic metastasis. The TNF-α-TNFR1 signalling pathway directly stimulates lymphatic endothelial cell activity through a VEGFR3-independent mechanism. However, VEGFR3-induced lymphatic endothelial cell tips are a prerequisite for lymphatic vessel growth in vivo , and a VEGFR3 blockade completely ablates TNF-α-induced lymphangiogenesis. Moreover, TNF-α-TNFR1-activated inflammatory macrophages produce high levels of VEGF-C to coordinately activate VEGFR3. Genetic deletion of TNFR1 ( Tnfr1 −/− ) in mice or depletion of tumour-associated macrophages (TAMs) virtually eliminates TNF-α-induced lymphangiogenesis and lymphatic metastasis. Gain-of-function experiments show that reconstitution of Tnfr1 +/+ macrophages in Tnfr1 −/− mice largely restores tumour lymphangiogenesis and lymphatic metastasis. These findings shed mechanistic light on the intimate interplay between inflammation and lymphangiogenesis in cancer metastasis, and propose therapeutic intervention of lymphatic metastasis by targeting the TNF-α-TNFR1 pathway. Among known pro-inflammatory cytokines, the tumour necrosis factor-alpha (TNF-α) and its receptors (TNFRs) are one of the best-characterized pro-inflammatory signalling pathways in the context of cancer and other pathological conditions. TNF-α is a multifunctional pro-inflammatory cytokine that regulates multifarious processes including inflammation, cellular apoptosis, coagulation, metabolism, insulin sensitivity, tumour growth and invasion, and vascular functions [1] , [2] , [3] , [4] . TNF-α carries out its biological functions by activation of TNFR1 and TNFR2, which are expressed in various cell types [5] , [6] . While TNFR1 is ubiquitously expressed in most human tissues and serves as a major signalling receptor for TNF-α, TNFR2 is restrictively expressed in immune cells and mediates limited biological functions [7] , [8] . Among all known functions, TNF-α is best known for its potent pro-inflammatory and apoptotic effects, involving activation of caspases and transcription factors, including nuclear factor-kappaB and activation protein-1 (ref. 9 ). Inflammation and lymphangiogenesis are tightly linked and inseparable processes under various pathological conditions [10] , [11] . Tissue oedema represents one of the cardinal signs of inflammatory disease with clinical significance, owing to excessive plasma leakage from the inflamed vasculatures relative to the limited drainage capacity of lymphatics in a given tissue [12] . As a compensatory mechanism, lymphangiogenesis is often triggered during acute and chronic inflammatory responses to reduce interstitial fluid pressure by enhancing the drainage capacity [13] . In contrast, impairment of drainage functions owing to defective lymphatics caused by infection, genetic alterations, trauma and surgical intervention would exacerbate the inflammation-associated tissue oedema. Consistent with this view, accumulating experimental evidence shows that stimulation of lymphangiogenesis is associated with beneficial effects in several preclinical acute and chronic inflammation models [14] , [15] , [16] , [17] , [18] . The vascular endothelial growth factor (VEGF)-C-VEGF receptor 3 (VEGFR3) signalling as the key lymphangiogenic pathway is crucially involved in inflammatory lymphangiogenesis [13] . TNF-α has recently been reported to mediate blood and lymphatic vessel remodelling in a mouse airway inflammation model [19] . TNF-α has also been reported to inhibit lymphatic endothelial cell (LEC) proliferation [20] , whereas the opposing effect of TNF-α in combination with angiopoietin-2 on LEC proliferation was also reported [21] . Despite these findings, the role of TNF-α in promoting lymphatic metastasis in mouse and human tumours remains completely unknown. Epithelial tumours often metastasize to regional lymph nodes and lymphatic metastasis in certain cancer types such as breast cancer, which is considered the most common route of metastasis [10] . Despite current knowledge of tumour inflammation, pro-inflammatory cytokines and lymphatic metastasis, little is known how tumour inflammation regulates tumour lymphangiogenesis and lymphatic metastasis. Moreover, reciprocal interplay between various pro-inflammatory cytokines and lymphangiogenic factors, which are frequently expressed at high levels in relation to tumour lymphangiogenesis and metastasis, remains largely unknown. In this study, we provide mechanistic evidence that the TNF-α-TNFR1 signalling coordinates with the VEGF-C-VEGFR3 signalling pathway in promoting lymphangiogenesis, which is crucial for lymphatic metastasis. Further, TNF-α-activated tumour-associated macrophages (TAMs) mediate tumour lymphangiogenesis and lymphatic metastasis by orchestrating the VEGF-C-VEGFR3 signalling system. Both loss-of-function and gain-of-function experiments together with pharmacological invention approaches demonstrate that targeting TAMs and the TNF-α-TNFR1 pro-inflammatory signalling is important for treatment of lymphatic metastasis. TNFR1 mediates direct effects of TNF-α-induced LEC activity To study the direct role of TNF-α in modulation of lymphangiogenesis, immortalized human LECs (hLECs) and primary mouse LECs (mLECs) [22] were stimulated with TNF-α in vitro . The mLECs expressed LEC-specific markers including LYVE-1 and Prox-1 ( Supplementary Fig. 1a ), a nuclear transcription factor. Interestingly, incubation of hLECs with TNF-α resulted in an elongated morphological change with spindle-like processes and actin reorganization ( Fig. 1a,b ). Similar to hLECs, TNF-α induced marked morphological changes with elongated spindle-like structures in mLECs ( Supplementary Fig. 1 ). TNF-α-induced LEC morphological changes were markedly different from those of VEGF-C-stimulated LECs ( Fig. 1a,b ). Quantification analysis showed that more than 90% of TNF-α-stimulated LECs underwent morphological changes, whereas VEGF-C-stimulated hLECs lacked such an overt effect ( Fig. 1a,b ). Consistent with morphological changes and actin reorganization, TNF-α potently stimulated hLEC migration that was equally robust to VEGF-C-induced cell motility ( Fig. 1a ). Similarly, TNF-α stimulated mLEC migration in vitro ( Supplementary Fig. 1d,e ). In support of its direct effect on LECs, stimulation of hLECs with TNF-α resulted in activation of phospholipase C γ1 (PLC-γ1), a known downstream component of TNF-α-triggered signalling [23] ( Fig. 1c ). Further, the GTP-bound activated Rac1 and CDC42 proteins, involved in actin reorganization and cell motility, were markedly activated in LECs by TNF-α, but not by VEGF-C, stimulation ( Fig. 1b ), supporting its direct effects on cell shape changes and migration. 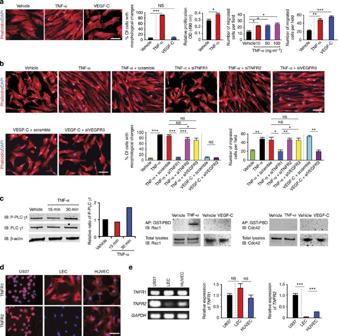Figure 1: TNFR expression and biological effects of TNF-α on LECs. (a) Morphology of immortalized hLECs. hLEC were stimulated with TNF-α, VEGF-C for 48 h followed by double staining with phalloidin (red) and 4',6-diamidino-2-phenylindole (DAPI; nuclei in blue). Vehicle-treated hLECs served as a control (vehicle). Scale bar, 100 μm. Quantification of LECs with elongated cell morphologies (six randomized fields × three independent samples per group). Quantification of TNF-α- and vehicle-treated LEC proliferation (six samples per group). Quantification of hLEC migration after treatment with various doses of TNF-α and vehicles (six samples per group). Quantification of TNF-α-, VEGF-C- and vehicle-treated hLEC migration (six samples per group). (b) Phalloidin (red) and DAPI (nuclei in blue) double immunostaining of TNF-α-, VEGF-C- or vehicle-treated hLECs in the presence or absence of scramble,TNFR1,TNFR2andVEGFR3siRNA. Scale bar, 100 μm. Quantification of indicated groups of LECs with elongated cell morphologies (six randomized fields × three independent samples per group). Quantification of indicated groups of LECs migration (six samples per group). (c) Western blot of phosphorylated PLCγ1 in vehicle- or 100 ng ml−1TNF-α-treated hLECs. β-Actin levels were used as standard control. Quantifications of densitometric ratio using β-actin for normalization. Pull-down assay of untreated or TNF-α-treated hLECs. Total and activated Cdc42 and Rac1 were detected using total and PAK-1 PBD affinity-purified (AP) cell lysates from vehicle-, TNF-α- or VEG-F-C-treated hLECs. (d) Immunostaining of TNFR1 and TNFR2 expression in U937 monocytes, hLECs and HUVECs. Cells were detected by double staining with TNFR1 (red)/DAPI (nuclei in blue) or TNFR2 (red)/DAPI (nuclei in blue). Scale bar, 100 μm. (e) RT–PCR and qPCR quantification ofTNFR1andTNFR2expression in U937 monocytes, hLECs and HUVECs. *P<0.05; **P<0.01; ***P<0.001; NS, not significant. All error bars represent s.e.m. AllPvalues were analysed according to Student’st-test. Figure 1: TNFR expression and biological effects of TNF-α on LECs. ( a ) Morphology of immortalized hLECs. hLEC were stimulated with TNF-α, VEGF-C for 48 h followed by double staining with phalloidin (red) and 4',6-diamidino-2-phenylindole (DAPI; nuclei in blue). Vehicle-treated hLECs served as a control (vehicle). Scale bar, 100 μm. Quantification of LECs with elongated cell morphologies (six randomized fields × three independent samples per group). Quantification of TNF-α- and vehicle-treated LEC proliferation (six samples per group). Quantification of hLEC migration after treatment with various doses of TNF-α and vehicles (six samples per group). Quantification of TNF-α-, VEGF-C- and vehicle-treated hLEC migration (six samples per group). ( b ) Phalloidin (red) and DAPI (nuclei in blue) double immunostaining of TNF-α-, VEGF-C- or vehicle-treated hLECs in the presence or absence of scramble, TNFR1 , TNFR2 and VEGFR3 siRNA. Scale bar, 100 μm. Quantification of indicated groups of LECs with elongated cell morphologies (six randomized fields × three independent samples per group). Quantification of indicated groups of LECs migration (six samples per group). ( c ) Western blot of phosphorylated PLCγ1 in vehicle- or 100 ng ml −1 TNF-α-treated hLECs. β-Actin levels were used as standard control. Quantifications of densitometric ratio using β-actin for normalization. Pull-down assay of untreated or TNF-α-treated hLECs. Total and activated Cdc42 and Rac1 were detected using total and PAK-1 PBD affinity-purified (AP) cell lysates from vehicle-, TNF-α- or VEG-F-C-treated hLECs. ( d ) Immunostaining of TNFR1 and TNFR2 expression in U937 monocytes, hLECs and HUVECs. Cells were detected by double staining with TNFR1 (red)/DAPI (nuclei in blue) or TNFR2 (red)/DAPI (nuclei in blue). Scale bar, 100 μm. ( e ) RT–PCR and qPCR quantification of TNFR1 and TNFR2 expression in U937 monocytes, hLECs and HUVECs. * P <0.05; ** P <0.01; *** P <0.001; NS, not significant. All error bars represent s.e.m. All P values were analysed according to Student’s t -test. Full size image We next analysed TNFR1 and TNFR2 expression in hLECs. Interestingly, TNFR1 was predominately expressed in hLECs, whereas these cells primarily lacked TNFR2 expression ( Fig. 1d ). Consistently, prominent expression of TNFR1 was also detected in mLECs by immunohistochemistry and western immunoblotting analyses ( Supplementary Fig. 1b,c ). In contrast, human umbilical vein endothelial cells (HUVECs) expressed similar levels of TNFR1 and TNFR2 ( Fig. 1d ). As a positive control, human U973 monocytes expressed high levels of TNFR1 and TNFR2 ( Fig. 1d ). These localization findings were validated by reverse transcription PCR (RT–PCR) and quantitative PCR (qPCR), confirming that LECs predominately expressed TNFR1 but lacked TNFR2 expression ( Fig. 1e ). To functionally associate TNFRs with TNF-α-stimulated LEC morphological changes and migration, we took a small interfering RNA (siRNA)-knockdown approach in our in vitro studies. Specific siRNA targeting TNFR1 virtually blocked TNF-α-induced cell shape changes ( Fig. 1b ). Similarly, the TNFR1 -specific siRNA completely inhibited TNF-α-stimulated LEC migration ( Fig. 1b ). In contrast, a scrambled siRNA and a siRNA specifically targeting TNFR2 had no effects on TNF-α-stimulated LEC morphological changes and migration ( Fig. 1b ). Since the VEGFR3 signalling has been described as the key pathway for lymphangiogenesis [24] , we next investigated whether TNF-α-stimulated LEC activity was dependent on the VEGFR3 signalling. TNF-α-stimulated LEC migration and morphological changes occurred in a VEGFR3-independent manner, since a VEGFR3 -specific siRNA had no effect on TNF-α-stimulated cells but effectively inhibited VEGF-C-induced LEC migration ( Fig. 1b ). Additional evidence was provided by incubation with an anti-mouse VEGFR3-specific neutralizing antibody in TNF-α-stimulated mLECs, showing no effects of anti-VEGFR3 on cell morphology and migration ( Supplementary Fig. 1d,e ). These findings demonstrate that TNF-α directly stimulates LEC migration and cell shape changes through a TNFR1-triggered signalling pathway, which is independent from the VEGFR3 signalling. TNF-α stimulates lymphangiogenesis in vivo Knowing the direct stimulatory effects of TNF-α on LECs in vitro , we next tested its ability in stimulation of lymphangiogenesis in vivo . We chose the mouse corneal lymphangiogenesis model because the cornea is an avascular tissue that lacks preexisting blood and lymphatic vessels [25] . Consistent with its in vitro LEC activity, implantation of TNF-α protein together with a slow-release polymer potently stimulated LYVE-1 + lymphatic vessel growth ( Fig. 2a ). TNF-α-induced lymphatic vessels appeared as a well-structured lymphatic network that grew from collecting limbal lymphatics towards the implanted micropellets ( Fig. 2a ). Of note, TNF-α-induced lymphatic growth appeared at the leading front of the vascular growth cone where blood microvessels were left behind. Interestingly, TNF-α-induced corneal lymphatic vessels were surrounded with a high number of CD206 + macrophages ( Supplementary Fig. 2 ). These findings demonstrate that TNF-α-stimulated lymphatic vessels develop through mechanisms that are independent from blood vessels. Similar to lymphangiogenesis, TNF-α, in this in vivo mouse model, also potently induced blood vessel formation, which was comparable to VEGF-C-induced angiogenesis ( Fig. 2a ). In concordance with its lymphangiogenic activity, distribution studies demonstrated that newly formed corneal lymphatics also expressed TNFR1 that were co-localized with LYVE-1 + structures ( Fig. 2b ). These findings indicate that TNF-α potently stimulated lymphangiogenesis in vivo , possibly through the TNFR1-mediated signalling. 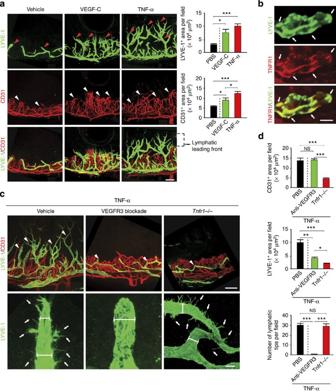Figure 2: TNF-α induces TNFR1-dependent corneal lymphangiogenesis. (a) Confocal images of TNF-α-, VEGF-C- and vehicle-induced LYVE-1+lymphangiogenesis (green) and CD31+angiogenesis (red) in mouse corneas. Red arrowheads indicate lymphatic vessels; white arrowheads indicate blood vessels. Scale bar, 200 μm. Quantification of corneal CD31+blood angiogenic and LYVE-1+lymphangiogenic vessels (n=4 mice per group). (b) High magnification of LYVE-1+(green) lymphangiogenic vessels that were co-stained with TNFR1 (red). Arrows point LYVE-1 and TNFR1 double-positive structures. Scale bar, 10 μm. (c) Confocal images of LYVE-1+lymphangiogenesis (green) and CD31+angiogenesis (red) in mouse corneas. TNF-α-induced angiogenesis and lymphangiogenesis inTnfr1−/−mice and in an anti-VEGFR3 neutralizing antibody-treated wild type (wt) mice were shown. Vehicle-treated mice served as a control. Arrowheads in upper panels indicate lymphatic vessels; arrows in lower panels point to filopodia tips sprouting from angiogenic lymphatic vessels. The diameters of lymphatic vessels are indicated. Scale bar, 200 μm (upper panels); 20 μm (lower panels). (d) Quantification of TNF-α-induced corneal CD31+angiogenesis and LYVE-1+lymphangiogenesis inTnfr1−/−mice, in VEGFR3 blockade-treatedwtmice and in vehicle-treatedwtmice (n=4 mice per group). *P<0.05; **P<0.01; ***P<0.001; NS, not significant. All error bars represent s.e.m. AllPvalues were analysed according to Student’st-test. Figure 2: TNF-α induces TNFR1-dependent corneal lymphangiogenesis. ( a ) Confocal images of TNF-α-, VEGF-C- and vehicle-induced LYVE-1 + lymphangiogenesis (green) and CD31 + angiogenesis (red) in mouse corneas. Red arrowheads indicate lymphatic vessels; white arrowheads indicate blood vessels. Scale bar, 200 μm. Quantification of corneal CD31 + blood angiogenic and LYVE-1 + lymphangiogenic vessels ( n =4 mice per group). ( b ) High magnification of LYVE-1 + (green) lymphangiogenic vessels that were co-stained with TNFR1 (red). Arrows point LYVE-1 and TNFR1 double-positive structures. Scale bar, 10 μm. ( c ) Confocal images of LYVE-1 + lymphangiogenesis (green) and CD31 + angiogenesis (red) in mouse corneas. TNF-α-induced angiogenesis and lymphangiogenesis in Tnfr1 −/− mice and in an anti-VEGFR3 neutralizing antibody-treated wild type ( wt ) mice were shown. Vehicle-treated mice served as a control. Arrowheads in upper panels indicate lymphatic vessels; arrows in lower panels point to filopodia tips sprouting from angiogenic lymphatic vessels. The diameters of lymphatic vessels are indicated. Scale bar, 200 μm (upper panels); 20 μm (lower panels). ( d ) Quantification of TNF-α-induced corneal CD31 + angiogenesis and LYVE-1 + lymphangiogenesis in Tnfr1 −/− mice, in VEGFR3 blockade-treated wt mice and in vehicle-treated wt mice ( n =4 mice per group). * P <0.05; ** P <0.01; *** P <0.001; NS, not significant. All error bars represent s.e.m. All P values were analysed according to Student’s t -test. Full size image TNF-α-stimulated VEGFR3-dependent lymphangiogenesis To study the functional relation between TNF-α-TNFR1-induced lymphangiogenesis and the VEGFR3 signalling pathway, we took two independent approaches. First, we used Tnfr1 −/− mice that completely lacked TNFR1. TNF-α-stimulated lymphangiogenesis was completely abrogated in Tnfr1 −/− mice ( Fig. 2c,d ), concluding that TNFR1 is functionally required for TNF-α-stimulated lymphangiogenesis. In contrast, VEGF-C-induced lymphangiogenesis in Tnfr1 −/− mice was not affected ( Supplementary Fig. 2 ), supporting the fact that VEGF-C directly stimulates lymphangiogenesis via VEGFR3 signalling. Second, we delivered a well-characterized anti-mouse VEGFR3 neutralizing antibody (VEGFR3 blockade) [22] , [26] to TNF-α-implanted mice. VEGFR3 blockade virtually inhibited TNF-α-stimulated lymphangiogenesis without affecting TNF-α-stimulated angiogenesis ( Fig. 2c,d ). High-magnification analysis of lymphatic vessels in various treated and non-treated groups showed the existence of fundamental differences of lymphatic structures in Tnfr1 −/− and VEGFR3-treated mice, although both groups showed attenuated phenotypes of TNF-α-stimulated lymphangiogenesis ( Fig. 2c ). In the Tnfr1 −/− mice, the resident limbal lymphatics possessed high numbers of LEC tips, whereas the VEGFR3 blockade-treated limbal lymphatic completely lacked LEC tips ( Fig. 2c,d ). Moreover, VEGFR3 blockade-treated lymphatics contained a high density of LECs at the leading front, resulting in enlarged tip-less lymphatic sprouts by accumulating LECs without formation of vascular networks ( Fig. 2c ). This type of enlarged lymphatic leading fronts most likely represents the consequence of lacking guidance by lymphatic growth factors. In addition to impairment of lymphangiogenesis, Tnfr1 −/− mice also exhibited impaired angiogenesis, suggesting that TNFR1 is essentially required for TNF-α-induced lymphangiogenesis and angiogenesis. TNF-α-dependent lymphatic metastasis in human tumours TNF-α is often expressed at high levels in human tumours and its potent lymphangiogenic activity seen in mouse corneal models promoted us to study its role in promoting lymphangiogenesis in human tumours. For clinical relevance, we chose TNF-α high and low natural expressing human ovarian cancers in our study because ovarian cancers frequently metastasize to regional lymph nodes [27] . OVCAR-8 and IGROV-1 human ovarian cancers have been previously characterized as TNF-α low- and high-expressing tumours [28] . In support of this notion, measurement of TNF-α protein in the conditioned media confirmed that IGROV-1 tumour cells produced approximately a 2.5-fold-higher amount of TNF-α relative to OVCAR-8 cells ( Fig. 3a ). Interestingly, IGROV-1 tumours contained a relatively high density of intratumoral lymphatics, whereas intratumoral lymphatics were barely detectable in OVCAR-8 tumours ( Fig. 3b ). These findings suggest that TNF-α is likely to contribute to tumour lymphangiogenesis. Consistent with its angiogenic function, vessel density in IGROV-1 tumours was higher than that in OVCAR-8 tumours ( Supplementary Fig. 3 ). 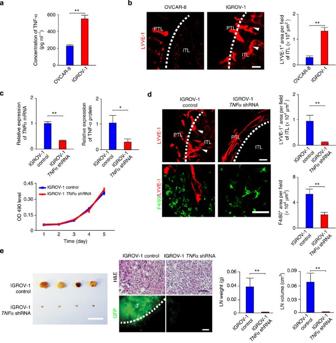Figure 3: TNF-α in human tumour lymphangiogenesis and metastasis. (a) ELISA assay of TNF-α protein levels in the conditioned medium of human OVCAR-8 and IGROV-1 ovarian cancer cells. (b) Confocal image of LYVE-1+tumour lymphatic vessels (red) in OVCAR-8 and IGROV-1 tumours. Dashed line marks the borders between tumour tissues and neighbouring healthy tissues. Arrowheads point to intratumoral lymphatics. Intratumoral lymphatic vessels were quantified (eight randomized fields per group). PTL, peritumoral lymphatics; ITL, intratumoral lymphatics. Scale bar, 100 μm. (c)TNFαshRNA inhibited TNF-α mRNA and protein expression in stably transfected IGROV-1 tumour cells (n=3 samples per group). Real-time PCR and ELISA were used for detection. Growth rates ofTNFαshRNA- and scrambled shRNA-transfected IGROV-1 cells. (d) Lymphatic vessel (red) localization and quantification inTNFαshRNA-transfected and control IGROV-1 tumours. Dashed line marks the borders between tumour tissues and neighbouring healthy tissues. Arrowheads point to intratumoral lymphatics. Lymphatic vessels were quantified from eight randomized fields per group. Localization and quantification of TAMs (green) inTNFαshRNA-transfected and control IGROV-1 tumours. Macrophages were quantified from eight randomized fields of six samples per group. Scale bar, 100 μm (upper panels); 50 μm (lower panels). (e) Left: representative sentinel lymph nodes (LNs) ofTNFαshRNA-transfected and control IGROV-1 tumour-bearing mice. Scale bar, 1 cm. Middle: hematoxylin and eosin stain (H&E) and fluorescence images of LNs.TNFαshRNA-transfected IGROV-1 metastases were detected in LNs. Dashed line marks the rim of a metastatic tumour in LN. T, tumour. Scale bar, 50 μm (upper panels); 100 μm (lower panels). Right: quantification of LN volume and weight inTNFαshRNA-transfected and control IGROV-1 tumour-bearing mice (n=10 mice per group). *P<0.05; **P<0.01. All error bars represent s.e.m. AllPvalues were analysed according to Student’st-test. Figure 3: TNF-α in human tumour lymphangiogenesis and metastasis. ( a ) ELISA assay of TNF-α protein levels in the conditioned medium of human OVCAR-8 and IGROV-1 ovarian cancer cells. ( b ) Confocal image of LYVE-1 + tumour lymphatic vessels (red) in OVCAR-8 and IGROV-1 tumours. Dashed line marks the borders between tumour tissues and neighbouring healthy tissues. Arrowheads point to intratumoral lymphatics. Intratumoral lymphatic vessels were quantified (eight randomized fields per group). PTL, peritumoral lymphatics; ITL, intratumoral lymphatics. Scale bar, 100 μm. ( c ) TNFα shRNA inhibited TNF-α mRNA and protein expression in stably transfected IGROV-1 tumour cells ( n =3 samples per group). Real-time PCR and ELISA were used for detection. Growth rates of TNFα shRNA- and scrambled shRNA-transfected IGROV-1 cells. ( d ) Lymphatic vessel (red) localization and quantification in TNFα shRNA-transfected and control IGROV-1 tumours. Dashed line marks the borders between tumour tissues and neighbouring healthy tissues. Arrowheads point to intratumoral lymphatics. Lymphatic vessels were quantified from eight randomized fields per group. Localization and quantification of TAMs (green) in TNFα shRNA-transfected and control IGROV-1 tumours. Macrophages were quantified from eight randomized fields of six samples per group. Scale bar, 100 μm (upper panels); 50 μm (lower panels). ( e ) Left: representative sentinel lymph nodes (LNs) of TNFα shRNA-transfected and control IGROV-1 tumour-bearing mice. Scale bar, 1 cm. Middle: hematoxylin and eosin stain (H&E) and fluorescence images of LNs. TNFα shRNA-transfected IGROV-1 metastases were detected in LNs. Dashed line marks the rim of a metastatic tumour in LN. T, tumour. Scale bar, 50 μm (upper panels); 100 μm (lower panels). Right: quantification of LN volume and weight in TNFα shRNA-transfected and control IGROV-1 tumour-bearing mice ( n =10 mice per group). * P <0.05; ** P <0.01. All error bars represent s.e.m. All P values were analysed according to Student’s t -test. Full size image To validate the lymphangiogenic function of TNF-α in these naturally occurring human ovarian cancers, TNFα -specific short hairpin RNA (shRNA)-knockdown experiments were performed in IGROV-1 tumours. As expected, stable transfection of TNFα- specific shRNA into IGROV-1 cells effectively suppressed TNFα mRNA and protein production without affecting tumour cell growth rates compared with the scrambled shRNA-transfected control tumour cells ( Fig. 3c ). Interestingly, TNFα -specific shRNA-transfected IGROV-1 tumours lacked intratumoral lymphatic vessels and only a barely detectable number of lymphatics existed in surrounding regions compared with the control tumours ( Fig. 3d ). Consistent with tumour lymphangiogenesis, IGROV-1 tumours frequently metastasized to lymph nodes and knockdown of TNFα by shRNA markedly suppressed lymphatic metastasis via inhibition of tumoral lymphangiogenesis ( Fig. 3e ). These data provide compelling evidence that TNF-α significantly contributes to tumour lymphangiogenesis and lymphatic metastasis. In addition to suppression of tumour lymphangiogenesis, TNFα shRNA also markedly inhibited infiltration of TAMs in tumours ( Fig. 3d ), consistent with the known inflammatory function of TNF-α. Taken together, our data demonstrate that TNF-α, in clinically relevant human tumour models, contributes to tumour lymphangiogenesis. TNF-α stimulates tumour lymphangiogenesis in mouse models We next investigated the capacity of TNF-α in stimulation of tumour lymphangiogenesis and metastasis in mouse tumour models. Mouse Lewis lung carcinoma (LLC) were genetically propagated to stably express human TNF-α and subcutaneously implanted to the syngeneic C57Bl/6 mice. Quantification analysis showed that TNF-α-transfected cells expressed ~8.5 ng ml −1 TNF-α that were secreted in the conditioned medium ( Supplementary Fig. 4a ). Despite production of TNF-α, the growth rate of the TNF-α-transfected cells was virtually identical to that of vector-transfected LLC cells ( Supplementary Fig. 4b ), demonstrating that TNF-α expression did not affect LLC tumour cell growth in vitro . TNF-α- and vector-transfected LLC tumours were stained with LYVE-1 for detection of peritumoral and intratumoral lymphatic vessels. Notably, TNF-α-expressing tumours contained an exceptionally high density of LYVE-1 + lymphatic vessels, which appeared as disorganized lymphatic networks ( Fig. 4a ). In addition, peritumoral lymphatics became highly dilated in the surrounding area of enhanced green fluorescent protein (EGFP)-positive TNF-α-expressing tumours ( Fig. 4a ). EGFP + tumour cells often existed in peritumoral lymphatics surrounding TNF-α-expressing tumours, indicating dissemination into the lymphatic system. In marked contrast, the vector-transfected control tumours completely lacked LYVE-1 + intratumoral lymphatics and the peritumoral lymphatics did not show overt dilation ( Fig. 4a ). Quantification analysis demonstrated that both intratumoral and peritumoral lymphatic vessel areas were markedly increased in TNF-α-expressing LLC tumours ( Fig. 4a ). These findings show that TNF-α potently induces tumour lymphangiogenesis. 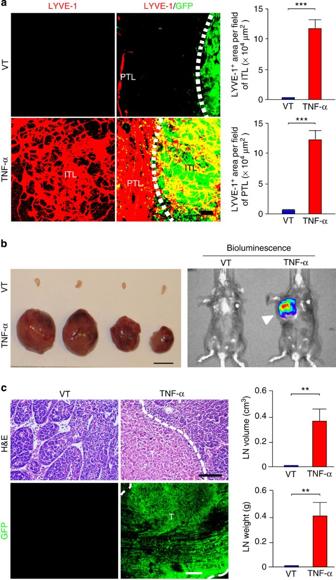Figure 4: TNF-α in mouse tumour lymphangiogenesis and metastasis. (a) Confocal image of vector or TNF-α-overexpressing LLC tumours. Overexpression of TNF-α in LLC tumours promoted peritumoral and intratumoral lymphangiogenesis (red LYVE-1 signals). Dashed line marks tumour borders, and LLC tumour cells expressed EGFP (green). ITL, intratumoral lymphatics; PTL, peritumoral lymphatics; VT, vector transfected. Scale bar, 100 μm. Quantification of peritumoral and intratumoral LYVE-1+lymphatics in TNF-α-overexpressing and vector-transfected LLC tumours (eight randomized fields per group). (b) Left: representative LNs of TNF-α- and vector-expressing LLC tumour-bearing mice. Scale bar, 5 mm. Right: a representative bioluminescence picture of mice that showed luciferase+TNF-α- and vector-expressing LLC tumour-bearing mice. Arrowhead indicates the metastatic LN. (c) Left: hematoxylin and eosin stain (H&E) and fluorescence images of LNs. TNF-α-expressing LLC metastases were detected in LNs. Dashed line marks the rim of a metastatic tumour in LN. T, tumour. Scale bar, 100 μm (upper panels); 100 μm (lower panels). Quantification of LN volume and weight in vector and TNF-α tumour-bearing mice (n=10 mice per group). **P<0.01; ***P<0.001. All error bars represent s.e.m. AllPvalues were analysed according to Student’st-test. Figure 4: TNF-α in mouse tumour lymphangiogenesis and metastasis. ( a ) Confocal image of vector or TNF-α-overexpressing LLC tumours. Overexpression of TNF-α in LLC tumours promoted peritumoral and intratumoral lymphangiogenesis (red LYVE-1 signals). Dashed line marks tumour borders, and LLC tumour cells expressed EGFP (green). ITL, intratumoral lymphatics; PTL, peritumoral lymphatics; VT, vector transfected. Scale bar, 100 μm. Quantification of peritumoral and intratumoral LYVE-1 + lymphatics in TNF-α-overexpressing and vector-transfected LLC tumours (eight randomized fields per group). ( b ) Left: representative LNs of TNF-α- and vector-expressing LLC tumour-bearing mice. Scale bar, 5 mm. Right: a representative bioluminescence picture of mice that showed luciferase + TNF-α- and vector-expressing LLC tumour-bearing mice. Arrowhead indicates the metastatic LN. ( c ) Left: hematoxylin and eosin stain (H&E) and fluorescence images of LNs. TNF-α-expressing LLC metastases were detected in LNs. Dashed line marks the rim of a metastatic tumour in LN. T, tumour. Scale bar, 100 μm (upper panels); 100 μm (lower panels). Quantification of LN volume and weight in vector and TNF-α tumour-bearing mice ( n =10 mice per group). ** P <0.01; *** P <0.001. All error bars represent s.e.m. All P values were analysed according to Student’s t -test. Full size image We next studied the possible functional properties of tumour-associated lymphatic vessels. We used the mouse ear tumour model, which was commonly used to assess lymphatic functions [29] . Vector and TNF-α tumours were implanted in the ears of mice and Indian ink was injected into tumours, and drainage of Indian ink could be visualized and quantified. Interestingly, the TNF-α tumour group contained a significantly higher number of visible lymphatics as compared with the control group ( Supplementary Fig. 4h ). These findings suggest that TNF-α-induced tumoral lymphatics are potentially functional. Consistent with this view, TNF-α tumours showed significantly lower tumour interstitial fluid pressure ( Supplementary Fig. 4i ). It should be emphasized that tumour blood vessels exhibited similar perfusion and permeability in both TNF-α and vector LLC tumours ( Supplementary Fig. 4j ). TNF-α stimulates sentinel lymph node metastasis To investigate whether TNF-α-induced intratumoral and peritumoral lymphatics could functionally mediate lymphatic metastasis, subcutaneous xenograft primary tumours were surgically removed. After 3–4 week post-tumour removal, a majority of TNF-α tumour-operated mice (60%) had visible and detectable metastases in sentinel lymph nodes ( Fig. 4b,c ). Lymphatic metastasis often occurred in bilateral sentinel lymph nodes. The presence of TNF-α-positive tumour tissues in lymph nodes was validated by histology and immunohistochemical detection of EGFP + tumour cells ( Fig. 4c ). Conversely, vector-transfected LLC tumour-bearing mice lacked obvious detectable lymph node metastasis ( Fig. 4b ). Similarly, histological detection did not show the presence of EGFP + tumour cells ( Fig. 4c ). Defective lymphangiogenesis and metastasis in Tnfr1 −/− mice Despite of hypervascularization, TNF-α-expressing tumours did not show accelerated growth rates ( Fig. 5a ), probably due to the high rate of tumour cell death in TNF-α tumours. To support of this notion, TNF-α-positive LLC tumours exhibited high rates of cellular apoptosis, necrosis and hypoxia, leading to large necrotic areas of tumour tissues ( Fig. 5b,c ; Supplementary Fig. 4c–g ). To study the functional impact of the TNF-α-TNFR1 signalling system on lymphangiogenesis and lymphatic metastasis, TNFR1 was genetically deleted in C57Bl/6 mice. TNFR-α-induced tumour lymphangiogenesis was completely ablated in Tnfr1 −/− mice ( Fig. 5d ). In addition to the complete lack of intratumoral lymphatic vessels, peritumoral lymphatic vessels were rarely detectable in TNF-α tumours growing in Tnfr1 −/− mice, which were indistinguishable from those of control tumours ( Fig. 5d ). Quantification analysis showed that both TNF-α-induced intratumoral and peritumoral lymphangiogenesis was completely abrogated by deletion of Tnfr1 −/− in mice and the basal level of detectable tumour lymphatics was indistinguishable from vector control tumours ( Fig. 5d ). These findings provide compelling evidence that TNFR1 is the functional receptor, which mediates TNF-α-induced tumour lymphangiogenesis. 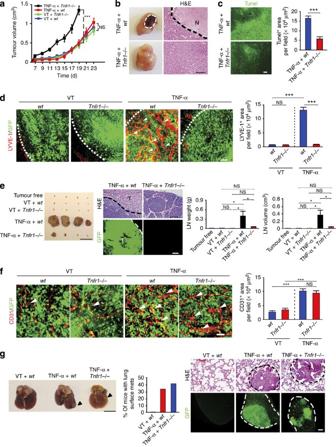Figure 5: Defective lymphangiogenesis and metastasis inTnfr1−/−mice. (a) Tumour growth rates of TNF-α- and vector-expressing LLC tumours implanted inwtandTnfr1−/−mice (n=12 mice per group). Tumour sizes were measured every other day and the experiments were terminated at day 23. (b) Gross appearance and hematoxylin and eosin stain (H&E) histology of TNF-α LLC tumours implanted inwtandTnfr1−/−mice. Dashed line marks the border between the necrotic and living tumour tissues. N, necrosis. Scale bar, 100 μm. (c) Tunel staining of TNF-α LLC tumours implanted inwtandTnfr1−/−mice and positive signals were quantified (12 randomized fields per group). Scale bar, 100 μm. (d) Primary TNF-α- and vector-expressing LLC tumours implanted inwtandTnfr1−/−mice were detected by LYVE-1 (red). LLC tumour cells expressed EGFP (green). Arrowheads point the lymphatic vessels. Scale bar, 100 μm. Quantification of LYVE-1+tumour lymphatics in TNF-α- and vector-expressing LLC tumours implanted inwtandTnfr1−/−mice (eight randomized fields per group). (e) Morphology of LNs of vector and TNF-α tumour-bearingwtandTnfr1−/−mice. Tumour-freewtmice served as a control. Scale bar, 1 cm. Histological examination of EGFP+metastasis in LNs (n=6 mice per group). Dashed line marks the border between a metastatic nodule and neighbouring LN tissues. T, tumour. Scale bar, 100 μm. Quantification of LN volume and weight in vector- and TNF-α tumour-bearingwtandTnfr1−/−mice (n=6 mice per group). (f) CD31+microvessels (red) and EGFP+tumour cells’ (green) double immunostaining of TNF-α- and vector-expressing LLC tumours implanted inwtandTnfr1−/−mice. Arrowheads point tumour blood vessels. Scale bar, 50 μm. Quantification of tumour CD31+angiogenic vessels inwtandTnfr1−/−mice (n=6 mice per group). (g) Left: representative lung morphology of vector tumour implanted inwtmice and TNF-α tumours implanted inwtandTnfr1−/−mice. Scale bar, 1 cm. Quantification of metastasis (n=12 mice per group). Right: lung histology of vector and TNF-α tumour-bearingwtandTnfr1−/−mice. Dashed line encircles the metastatic nodules. T, tumour. Scale bar, 100 μm (upper panels); 400 μm (lower panels). *P<0.05; ***P<0.001; NS, not significant. All error bars represent s.e.m. AllPvalues were analysed according to Student’st-test. d, days. Figure 5: Defective lymphangiogenesis and metastasis in Tnfr1 −/− mice. ( a ) Tumour growth rates of TNF-α- and vector-expressing LLC tumours implanted in wt and Tnfr1 −/− mice ( n =12 mice per group). Tumour sizes were measured every other day and the experiments were terminated at day 23. ( b ) Gross appearance and hematoxylin and eosin stain (H&E) histology of TNF-α LLC tumours implanted in wt and Tnfr1 −/− mice. Dashed line marks the border between the necrotic and living tumour tissues. N, necrosis. Scale bar, 100 μm. ( c ) Tunel staining of TNF-α LLC tumours implanted in wt and Tnfr1 −/− mice and positive signals were quantified (12 randomized fields per group). Scale bar, 100 μm. ( d ) Primary TNF-α- and vector-expressing LLC tumours implanted in wt and Tnfr1 −/− mice were detected by LYVE-1 (red). LLC tumour cells expressed EGFP (green). Arrowheads point the lymphatic vessels. Scale bar, 100 μm. Quantification of LYVE-1 + tumour lymphatics in TNF-α- and vector-expressing LLC tumours implanted in wt and Tnfr1 −/− mice (eight randomized fields per group). ( e ) Morphology of LNs of vector and TNF-α tumour-bearing wt and Tnfr1 −/− mice. Tumour-free wt mice served as a control. Scale bar, 1 cm. Histological examination of EGFP + metastasis in LNs ( n =6 mice per group). Dashed line marks the border between a metastatic nodule and neighbouring LN tissues. T, tumour. Scale bar, 100 μm. Quantification of LN volume and weight in vector- and TNF-α tumour-bearing wt and Tnfr1 −/− mice ( n =6 mice per group). ( f ) CD31 + microvessels (red) and EGFP + tumour cells’ (green) double immunostaining of TNF-α- and vector-expressing LLC tumours implanted in wt and Tnfr1 −/− mice. Arrowheads point tumour blood vessels. Scale bar, 50 μm. Quantification of tumour CD31 + angiogenic vessels in wt and Tnfr1 −/− mice ( n =6 mice per group). ( g ) Left: representative lung morphology of vector tumour implanted in wt mice and TNF-α tumours implanted in wt and Tnfr1 −/− mice. Scale bar, 1 cm. Quantification of metastasis ( n =12 mice per group). Right: lung histology of vector and TNF-α tumour-bearing wt and Tnfr1 −/− mice. Dashed line encircles the metastatic nodules. T, tumour. Scale bar, 100 μm (upper panels); 400 μm (lower panels). * P <0.05; *** P <0.001; NS, not significant. All error bars represent s.e.m. All P values were analysed according to Student’s t -test. d, days. Full size image We next studied the impact of deletion of Tnfr1 gene in mice on TNF-α-induced lymphatic metastasis. Consistent with lymphangiogenesis defects, TNF-α-induced sentinel lymph node metastasis was also largely attenuated in Tnfr1 −/− mice, although a small number of nodes still had metastatic lesions ( Fig. 5e ). Histological and immunohistochemical analyses confirmed the fact that most Tnfr1 −/− lymph nodes lacked metastatic lesions in both vector- and TNF-α tumour-bearing mice ( Fig. 5e ; Supplementary Fig. 5a ). These data validate the findings that TNFR1 is essentially required for TNF-α-induced lymphangiogenesis and lymphatic metastasis. On the basis of these findings, it is reasonably speculated that targeting TNFR1 signalling system would be crucial for treatment of TNF-α-promoted lymphatic metastasis. Abrogation of tumour lymphangiogenesis in Tnfr1 −/− mice Since TNF-α is also known to promote angiogenesis [30] , we investigated tumour angiogenesis in TNF-α and vector tumours. Interestingly, vascular density in TNF-α-expressing LLC tumours was markedly higher compared with that in vector control tumours ( Fig. 5f ; Supplementary Fig. 5b ). These CD31 + tumour blood microvessels were significantly smaller than LYVE-1 + lymphatic vessels and generally lacked VEGFR3 expression ( Supplementary Fig. 5b ). TNF-α tumours growing in Tnfr1 −/− mice resulted in an accelerated tumour growth rate rather than inhibition of tumour growth ( Fig. 5a ). Paradoxically, TNF-α-induced tumour angiogenesis was not affected in Tnfr1 −/− mice relative to those in wt mice ( Fig. 5f ), suggesting that TNFR1 is not critically required for TNFR1-induced tumour angiogenesis. In support of this view, a recent study demonstrates that TNFR2 is critically required for TNF-α-mediated physiological and pathological angiogenesis [31] . Accelerated TNF-α tumour growth rates without enhanced angiogenesis promoted us to study the death-related functions mediated by TNFR1. Interestingly, TNF-α-induced tumour cellular apoptosis and tumour tissue necrosis were markedly attenuated in Tnfr1 −/− mice compared with those in wt mice ( Fig. 5b ). These findings reconcile with TNFR1-mediated cell death in a variety of cell types including tumour cells. Thus, acceleration of TNF-α tumour growth rates in Tnfr1 −/− mice is likely due to reduction of tumour cell apoptosis and necrosis but not vascularization. This view is further supported by the fact that deletion of TNFR1 in mice did not affect vector control tumour growth rates ( Fig. 5a ). TNF-α-promoted TNFR1-independent bloodstream metastasis Alteration of angiogenesis by TNF-α promoted us to study bloodstream metastasis in wt and Tnfr1 −/− mice. Interestingly, more than 30% of TNF-α tumour-bearing mice contained visible pulmonary metastases in wt mice ( Fig. 5g ). These metastatic lesions could be histologically distinguished from the neighbouring healthy lung tissues and they expressed EGFP as a tumour cell marker ( Fig. 5g ). In contrast, no visible and microscopic pulmonary metastatic lesions were detectable in vector control tumour-bearing mice ( Fig. 5g ). These findings show that TNF-α promotes pulmonary metastasis in mouse tumour model. To study the role of TNFR1 in mediation of TNF-α-induced pulmonary metastasis, TNF-α-expressing tumours were implanted in Tnfr1 −/− mice. Notably, deletion of TNFR1 in mice did not affect TNF-α-induced lung metastasis, and a similar number of visible and microscopic metastatic lesions were present in wt and Tnfr1 −/− mice ( Fig. 5g ). Taken together, these findings show that TNF-α promotes bloodstream metastasis through TNFR1-independent mechanism. Inhibition of lymphangiogenesis and metastasis by anti-VEGFR3 To study the interactive relation of the TNF-α-TNFR1 system and VEGFR3 signalling in promoting tumour lymphangiogenesis and lymphatic metastasis, an anti-VEGFR3 neutralizing antibody [32] , [33] was used to treat TNF-α-expressing tumour-bearing mice. As expected, VEGFR3 blockade effectively blocked VEGF-C-induced tumour lymphangiogenesis, demonstrating the inhibitory effectiveness of the anti-VEGFR3 neutralizing antibody ( Fig. 6a ). In comparison with VEGF-C tumours, TNF-α-expressing tumours possessed a high number of exceptionally dilated peritumoral lymphatics ( Fig. 6a ). Strikingly, VEGFR3 blockade potently inhibited TNF-α-induced lymphangiogenesis, leading to complete ablation of intratumoral lymphangiogenesis ( Fig. 6a ). Detailed examination of lymphatic vessel structures revealed that VEGFR3 blockade completely inhibited the lymphatic endothelial tip cell formation in both VEGF-C and TNF-α tumours, whereas the vehicle-treated control VEGF-C and TNF-α tumours contained high numbers of lymphatic tips ( Fig. 6b ). Anti-VEGFR3-treated TNF-α tumours had a substantial number of peritumoral lymphatics that appeared as ‘mushroom-shaped’ structures with excessive accumulation of LECs without sprouting ( Fig. 6b ). Histological analysis showed that VEGFR3 blockade-treated enlarged lymphatic structures contained a similar number of Ki67 + proliferative LECs as those of vehicle-treated samples ( Supplementary Fig. 6 ). Thus, it is likely that both LEC proliferation and lymphatic dilation are involved in enlargement of VEGFR3 blockade-treated lymphatics. These tumour studies validate similar findings from the corneal lymphangiogenesis experiments ( Fig. 2a–d ). Consistent with inhibition of tumour lymphangiogenesis, VEGFR3 blockade potently suppressed TNF-α induced lymphatic metastasis ( Fig. 6c ). These findings demonstrate that TNF-α-stimulated lymphangiogenesis is completely dependent on the VEGFR3 signalling system. 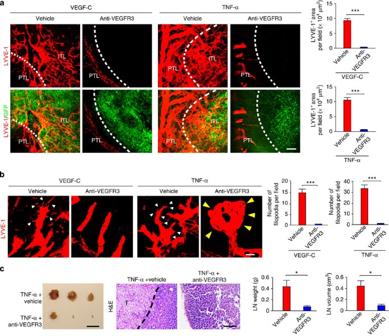Figure 6: Anti-VEGFR3 blocks TNF-α-lymphangiogenesis and metastasis. (a) Confocal images of VEGF-C- and TNF-α-overexpressing LLC tumours. VEGF-C and TNF-α tumour-bearing mice were treated with an anti-VEGFR3 neutralizing antibody. Peri- and intratumoral lymphatics (PTLs and ITLs) were detected with LYVE-1 (red), and tumour cells expressed EGFP (green). Dashed line marks borders between tumour and neighbouring tissues. Scale bar, 100 μm. Quantification of LYVE-1+lymphatic vessels in vehicle- and VEGFR3 blockade-treated VEGF-C and TNF-α tumours. Quantification data were obtained from eight randomized fields per group. (b) Confocal images of lymphatic vessels in VEGF-C- and TNF-α-overexpressing LLC tumours. Impairment of lymphatic tips of VEGF-C- and TNF-α-induced tumour lymphatic vessels by VEGFR3 blockade treatment. White arrowheads indicate sprouting lymphatic tips; yellow arrowheads indicate the ‘mushroom-like’ lymphatic structure without sprouting tips often seen in VEGFR3 blockade-treated TNF-α tumours. Scale bar, 100 μm. Quantification of lymphatic tips in vehicle- and VEGFR3 blockade-treated VEGF-C and TNF-α tumours. Quantification data were obtained from eight randomized fields per group. (c) Left: morphology (scale bar, 1 cm) and histological examination (scale bar, 100 μm) of LN. LNs of vehicle- and VEGFR3 blockade-treated TNF-α tumour-bearing mice were examined. Dashed line marks the border between a metastatic nodule and neighbouring LN tissues. T, tumour. Right: quantification of LN volume and weight of vehicle- and VEGFR3 blockade-treated TNF-α tumour-bearing mice (n=6 mice per group). *P<0.05; ***P<0.001. All error bars represent s.e.m. AllPvalues were analysed according to Student’st-test. H&E, hematoxylin and eosin stain. Figure 6: Anti-VEGFR3 blocks TNF-α-lymphangiogenesis and metastasis. ( a ) Confocal images of VEGF-C- and TNF-α-overexpressing LLC tumours. VEGF-C and TNF-α tumour-bearing mice were treated with an anti-VEGFR3 neutralizing antibody. Peri- and intratumoral lymphatics (PTLs and ITLs) were detected with LYVE-1 (red), and tumour cells expressed EGFP (green). Dashed line marks borders between tumour and neighbouring tissues. Scale bar, 100 μm. Quantification of LYVE-1 + lymphatic vessels in vehicle- and VEGFR3 blockade-treated VEGF-C and TNF-α tumours. Quantification data were obtained from eight randomized fields per group. ( b ) Confocal images of lymphatic vessels in VEGF-C- and TNF-α-overexpressing LLC tumours. Impairment of lymphatic tips of VEGF-C- and TNF-α-induced tumour lymphatic vessels by VEGFR3 blockade treatment. White arrowheads indicate sprouting lymphatic tips; yellow arrowheads indicate the ‘mushroom-like’ lymphatic structure without sprouting tips often seen in VEGFR3 blockade-treated TNF-α tumours. Scale bar, 100 μm. Quantification of lymphatic tips in vehicle- and VEGFR3 blockade-treated VEGF-C and TNF-α tumours. Quantification data were obtained from eight randomized fields per group. ( c ) Left: morphology (scale bar, 1 cm) and histological examination (scale bar, 100 μm) of LN. LNs of vehicle- and VEGFR3 blockade-treated TNF-α tumour-bearing mice were examined. Dashed line marks the border between a metastatic nodule and neighbouring LN tissues. T, tumour. Right: quantification of LN volume and weight of vehicle- and VEGFR3 blockade-treated TNF-α tumour-bearing mice ( n =6 mice per group). * P <0.05; *** P <0.001. All error bars represent s.e.m. All P values were analysed according to Student’s t -test. H&E, hematoxylin and eosin stain. Full size image Essential role of TAMs in lymphangiogenesis and metastasis As TNF-α is a potent pro-inflammatory cytokine, and inflammation and lymphangiogenesis are tightly linked two processes [10] , we therefore studied the involvement of inflammatory cells in lymphangiogenesis in the tumour microenvironment. As expected, TNF-α-expressing tumours contained an exceptionally high density of TAMs as detected by fluorescence-activated cell sorting (FACS) analysis and by immunohistochemistry staining ( Fig. 7a–c ). Moreover, most of these TAMs appeared to be the CD206 + subpopulations of TAMs ( Fig. 7b ). In vitro studies showed that TNF-α was able to directly induce monocyte migration ( Supplementary Fig. 7a ). In TNF-α tumours implanted in wt mice, Ccl2 expression level was higher than that in the vector tumours ( Supplementary Fig. 7b ). These findings suggest that both direct and indirect mechanisms are involved in mobilization of monocytes/macrophages in tumours by TNF-α. We next took two approaches to inhibit macrophage involvement in TNF-α-expressing tumour tissues. First, we implanted TNF-α-expressing tumour in Tnfr1 −/− mice, and interestingly, the number of TAMs was significantly decreased ( Fig. 7c ), suggesting that TNFR1 is involved in recruitment of TAMs. As described above, TNF-α-induced lymphangiogenesis was ablated in Tnfr1 −/− mice ( Fig. 7c ). We also used clodronate liposomes, a known agent for macrophage depletion [34] , which markedly inhibited TNF-α-induced TAMs ( Fig. 7c ). Clodronate liposomes treatment resulted in suppression of TNF-α-induced lymphangiogenesis ( Fig. 7c ). Consistent with the decrease of TAM numbers, clodronate liposome treatment markedly inhibited TNF-α-promoted lymphatic metastasis ( Fig. 7d,e ). These findings provide convincing evidence that TAMs are essentially required for mediation of TNF-α-induced lymphangiogenesis and lymphatic metastasis. 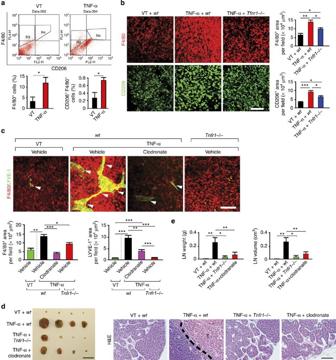Figure 7: TAMs mediate TNF-α-lymphangiogenesis and metastasis. (a) FACS analysis of the F4/80+pan population and F4/80+CD206+M2 subpopulation of TAMs in vector and TNF-α tumours (n=6 samples per group). (b) Immunohistochemical analysis of F4/80+(red) and CD206+TAMs (green) in TNF-α tumour-bearingwtandTnfr1−/−mice. Vector tumours implanted inwtmice served as a control. Scale bar, 100 μm. Quantification data were obtained from eight randomized fields per group. (c) Confocal images of TAMs and lymphangiogenesis in primary tumours. TAMs (red) and tumour lymphatic vessels (green) in clodronate liposome-treated TNF-α tumour-bearingwtmice. TAMs and lymphatics in TNF-α tumour-bearingTnfr1−/−mice were also analysed. Vector tumours served as a control. Arrowheads point to tumour lymphatic vessels. Scale bar, 100 μm. Quantification of tumour TAMs and LYVE-1+lymphatic vessels in various treated and non-treated groups. Quantification data were obtained from eight randomized fields per group. (d) Morphology (scale bar, 1 cm) and hematoxylin and eosin stain (H&E) histological staining (scale bar, 100 μm) of LNs from various treated and non-treated tumour-bearing mice. Dashed lines mark the border between metastatic tumour and LN tissues. T, tumour. (e) Quantification of LN volume and weight of various groups (n=6 mice per group). *P<0.05; **P<0.01; ***P<0.001. All error bars represent s.e.m. AllPvalues were analysed according to Student’st-test. Figure 7: TAMs mediate TNF-α-lymphangiogenesis and metastasis. ( a ) FACS analysis of the F4/80 + pan population and F4/80 + CD206 + M2 subpopulation of TAMs in vector and TNF-α tumours ( n =6 samples per group). ( b ) Immunohistochemical analysis of F4/80 + (red) and CD206 + TAMs (green) in TNF-α tumour-bearing wt and Tnfr1 −/− mice. Vector tumours implanted in wt mice served as a control. Scale bar, 100 μm. Quantification data were obtained from eight randomized fields per group. ( c ) Confocal images of TAMs and lymphangiogenesis in primary tumours. TAMs (red) and tumour lymphatic vessels (green) in clodronate liposome-treated TNF-α tumour-bearing wt mice. TAMs and lymphatics in TNF-α tumour-bearing Tnfr1 −/− mice were also analysed. Vector tumours served as a control. Arrowheads point to tumour lymphatic vessels. Scale bar, 100 μm. Quantification of tumour TAMs and LYVE-1 + lymphatic vessels in various treated and non-treated groups. Quantification data were obtained from eight randomized fields per group. ( d ) Morphology (scale bar, 1 cm) and hematoxylin and eosin stain (H&E) histological staining (scale bar, 100 μm) of LNs from various treated and non-treated tumour-bearing mice. Dashed lines mark the border between metastatic tumour and LN tissues. T, tumour. ( e ) Quantification of LN volume and weight of various groups ( n =6 mice per group). * P <0.05; ** P <0.01; *** P <0.001. All error bars represent s.e.m. All P values were analysed according to Student’s t -test. Full size image Macrophage-derived VEGF-C in lymphatic metastasis To further elucidate the role of TAMs in mediation of TNF-α-induced lymphangiogenesis and metastasis, TAMs were isolated. Interestingly, TAMs in TNF-α tumours expressed nearly a fourfold increase in Vegfc mRNA ( Fig. 8a ). Notably, Vegfc expression levels in TNF-α-induced TAMs were completely ablated in Tnfr1 −/− mice. In contrast to Vegfc , expression levels of Vegfd , another structurally related lymphangiogenic factor that binds to VEGFR3 [35] , were not increased in TNF-α-expressing tumours ( Fig. 8a ). Consistently, VEGF-C protein level is also upregulated in TAMs in TNF-α tumours ( Fig. 8a ). We next performed a functional rescue experiment in which F4/80 + cells isolated from blood of wt mice were transplanted into Tnfr1 −/− mice. Interestingly, transplantation of F4/80 + cells isolated from wt mice led to restoration of TNF-α-induced tumour lymphangiogenesis in Tnfr1 −/− mice ( Fig. 8b ). Although this approach only rescued ~40% of TNF-α-stimulated tumour lymphangiogenesis ( Fig. 8b ), these findings convincingly showed the crucial role of F4/80 + cells in mediation of TNF-α-induced tumour lymphangiogenesis. Notably, transplantation of F4/80 + cells isolated from wt mice promoted TNF-α-induced lymphatic metastasis in Tnfr1 −/− mice ( Fig. 8c ), indicating that monocytes are essentially involved in mediation of TNF-α-stimulated lymphatic metastasis. 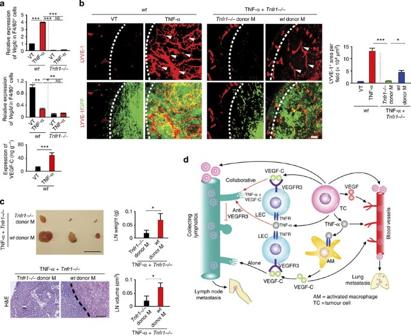Figure 8: Lymphangiogenesis inTnfr1−/−mice bywtF4/80+cells. (a) Quantitative PCR analysis ofVegfcandVegfdmRNA levels in TAMs isolated from vector and TNF-α tumour-bearingwtandTnfr1−/−mice (n=6 samples per group). ELISA analysis of VEGF-C protein levels in TAMs isolated from vector and TNF-α tumours (n=3 samples per group). (b) Confocal images of lymphatic vessels in TNF-α tumour-bearingTnfr1−/−mice that received transplantation of F4/80+cells isolated fromwtandTnfr1−/−mice. Intratumoral lymphatics were detected with LYVE-1 (red) and EGFP-expressing tumour cells (green). Arrowheads indicate intratumoral lymphatic vessels. Dashed line marks the tumour borders. Scale bar, 100 μm. Quantification of intratumoral LYVE-1+lymphatic vessels. Quantification data were obtained from eight randomized fields per group. (c) Morphology (scale bar, 1 cm) and hematoxylin and eosin stain (H&E) histological staining (scale bar, 100 μm) of LNs from TNF-α tumour-bearingTnfr1−/−mice that received transplantation of F4/80+cells isolated fromwtandTnfr1−/−mice. Dashed line marks the border between metastatic tumour and LN tissues. T, tumour. Quantification of LN volume and weight of various groups (n=6 mice per group). (d) Mechanistic diagram showing that TNF-α induced tumour inflammatory lymphangiogenesis and lymphatic metastasis by orchestrating the VEGF-C-VEGFR3 signalling. Tumour cell-derived TNF-α induces LEC proliferation and migration, and TNF-α-activated TAMs produce VEGF-C to induce lymphatic vessel tip cell formation. Both processes are crucial for the formation of a functional lymphatic network. Inhibition of the VEGFR3 signalling results in the formation of enlarged blind ends of preexisting lymphatics without sprouting. *P<0.05; **P<0.01; ***P<0.001; NS, not significant. All error bars represent s.e.m. AllPvalues were analysed according to Student’st-test. Figure 8: Lymphangiogenesis in Tnfr1 −/− mice by wt F4/80 + cells. ( a ) Quantitative PCR analysis of Vegfc and Vegfd mRNA levels in TAMs isolated from vector and TNF-α tumour-bearing wt and Tnfr1 −/− mice ( n =6 samples per group). ELISA analysis of VEGF-C protein levels in TAMs isolated from vector and TNF-α tumours ( n =3 samples per group). ( b ) Confocal images of lymphatic vessels in TNF-α tumour-bearing Tnfr1 −/− mice that received transplantation of F4/80 + cells isolated from wt and Tnfr1 −/− mice. Intratumoral lymphatics were detected with LYVE-1 (red) and EGFP-expressing tumour cells (green). Arrowheads indicate intratumoral lymphatic vessels. Dashed line marks the tumour borders. Scale bar, 100 μm. Quantification of intratumoral LYVE-1 + lymphatic vessels. Quantification data were obtained from eight randomized fields per group. ( c ) Morphology (scale bar, 1 cm) and hematoxylin and eosin stain (H&E) histological staining (scale bar, 100 μm) of LNs from TNF-α tumour-bearing Tnfr1 −/− mice that received transplantation of F4/80 + cells isolated from wt and Tnfr1 −/− mice. Dashed line marks the border between metastatic tumour and LN tissues. T, tumour. Quantification of LN volume and weight of various groups ( n =6 mice per group). ( d ) Mechanistic diagram showing that TNF-α induced tumour inflammatory lymphangiogenesis and lymphatic metastasis by orchestrating the VEGF-C-VEGFR3 signalling. Tumour cell-derived TNF-α induces LEC proliferation and migration, and TNF-α-activated TAMs produce VEGF-C to induce lymphatic vessel tip cell formation. Both processes are crucial for the formation of a functional lymphatic network. Inhibition of the VEGFR3 signalling results in the formation of enlarged blind ends of preexisting lymphatics without sprouting. * P <0.05; ** P <0.01; *** P <0.001; NS, not significant. All error bars represent s.e.m. All P values were analysed according to Student’s t -test. Full size image To further strengthen our findings on macrophage-derived VEGF-C in TNF-α-induced lymphangiogenesis, isolated mouse monocytes were stimulated with TNF-α. Stimulation of monocytes in vitro led to an activated morphological phenotype that showed high numbers of filopodia ( Supplementary Fig. 8a ). Consistent with morphological changes, TNF-α stimulated monocyte migration ( Supplementary Fig. 8a ). Interestingly, TNF-α-stimulated monocytes expressed a high level of VEGF-C mRNA, but not VEGF-D ( Supplementary Fig. 8b ). These in vitro data further validate our in vivo findings. We provide compelling experimental evidence showing that TNF-α, as one of the prominent pro-inflammatory cytokines, directly modulates LEC functions through activation of TNFR1 expressed in these cells. The TNF-α-TNFR1 lymphatic signalling pathway is completely dependent on the VEGFR3-mediated lymphatic tip formation to constitute a lymphatic network. To ensure the activation of the VEGFR3 signalling pathway, TNF-α recruits and activates inflammatory macrophages to produce high levels of one of the VEGFR3 ligands, VEGF-C. Thus, TNF-α regulates the VEGF-C-VEGFR3 pathway to promote lymphangiogenesis and the functional consequence of the interplay between two signalling pathways in the tumour microenvironment results in cancer metastasis to sentinel lymph nodes. While intratumoral lymphatics are well correlated with lymph node metastasis, the lymphatics in pathological tissues may lack appropriate functions as seen in ovarian cancers [36] . However, it is highly plausible that peritumoral lymphatics can also contribute to lymphatic metastasis. The other possibility is that the TNF-α-induced apoptotic and necrotic cellular debris could potentially activate a scavenger receptor on lymphatic vessels, leading to lymphangiogenesis and metastasis. These interesting issues related to functions of tumoral lymphatics warrant future studies. Our present study provides several novel and mechanistic insights underlying inflammation-mediated tumour invasion and metastasis. First, we show that TNF-α, a prominent pro-inflammatory cytokine, promotes lymphangiogenesis and lymphatic metastasis in a clinically relevant human and mouse epithelial carcinoma tumour models. Clinical studies show that elevated levels of TNF-α are present in a substantial number of cancer patients [37] and TNF-α contributes to malignant disease through several mechanisms: tumour inflammation, tumour angiogenesis, promoting epithelial–mesenchymal transition (EMT) and activation of matrix metalloproteinases (MMPs). Tumour-infiltrated host cells induce upregulation of an array of inflammatory targeted cytokines including TNF-α and interleukin-1β that induce tumour inflammation [38] . TAMs directly participate in tumour invasion and metastasis [39] . Alternatively, TAMs propagate the tumour microenvironment that promotes tumour growth and invasion. TNF-α exhibits potent pro-angiogenic activity and stimulates tumour angiogenesis [40] , which is essential for tumour growth and invasion. TNF-α induces EMT transition in epithelial carcinomas and thus promotes tumour invasion [41] , and promotes tumour invasion by activation of MMPs such as MMP9 (ref. 42 ). In a recent study, it has been shown that soluble and membrane-bound TNF-α may display opposing effects on tumour growth and tumour-associated myeloid cells [43] . Differential effects of soluble and membrane-bound TNF-α in lymphangiogenesis and metastasis warrant future studies. Despite broad reorganization of these functions in the tumour microenvironment, the role of this prominent pro-inflammatory cytokine in modulation of tumour lymphangiogenesis and lymphatic metastasis remains completely unknown. Here we show that isolated LECs directly express TNFR1 that mediates TNF-α-induced LEC motility in vitro . These in vitro findings have been validated using an in vivo corneal lymphangiogenesis [25] and tumour lymphangiogenesis models. Expression of TNFR2 is limited in HUVECs but not in LECs, indicating the distinctive functions of these two receptors in modulation of angiogenesis and lymphangiogenesis. An interesting finding in our work is that TNF-α-induced lymphangiogenesis can be completely blocked by anti-VEGFR3 neutralizing antibody. Why would VEGFR3 inhibition completely suppress the direct effect of TNF-α–induced lymphangiogenesis? In the cornea, we show that VEGFR3 blockade completely inhibits the LEC tip formation at leading front of TNF-α-induced lymphangiogenic vessels, resulting in the formation of large-diameter and blind-end lymphatics in the limbus. Expansion of the existing lymphatic vessels without sprouting is most likely caused by accumulation of TNF-α-stimulated LECs. This view is further supported in the tumour environment in which VEGFR3 inhibition completely prevents tip LEC formation in TNF-α-stimulated lymphatic vessels. At the growing cone of some of the VEGFR3 blockade-treated lymphatic vessels, TNF-α-induced tumour lymphatic sprouting is replaced by a ‘mushroom-shaped’ structure, which most likely represents accumulation of LECs owing to the direct proliferative and migratory effects of TNF-α. These findings suggest that TNF-α-mediated proliferative and migratory effects are necessary but not sufficient to trigger lymphatic vessel growth and the formation of a lymphatic network. VEGFR3-induced LEC tip formation is fundamentally required for sprouting and guidance of lymphatic vessel growth. Without VEGFR3-induced tip LEC formation, TNF-α only induces accumulation of LECs at the forefront of growing lymphatics, and is thus unable to induce lymphangiogenesis. A similar mechanism might also exist in other lymphangiogenic factor-induced lymphangiogenesis in the tumour environment. Recent supportive evidence from our lab shows that another direct lymphangiogenic factor, FGF-2, -induced lymphangiogenesis is also dependent on VEGFR3-mediated tip LEC formation [22] . If these findings can be generalized with other lymphangiogenic factors, the VEGFR3-mediated LEC tip cell formation is a common mechanism for various factor-induced lymphangiogenesis, with an exception of certainly direct lymphangiogenic factors such as VEGF-A, angiopoietin-2 and platelet-derived growth factor-BB (PDGF-BB) [33] , [44] , [45] , [46] . This conclusion reconciles with the general view of the essential role of the VEGFR3-mediated signalling in modulation of developmental lymphangiogenesis and pathological lymphangiogenesis in adults. To ensure persistent activation of VEGFR3, TNF-α, in the tumour microenvironment, recruits and activates macrophages, which produce high levels of VEGF-C, a prominent ligand for VEGFR3 (ref. 24 ). In contrast, VEGF-D, another VEGFR3 ligand, is not upregulated. It is unclear why VEGF-C and -D are differentially regulated in TNF-α-activated macrophages. In an airway inflammation mouse model, TNF-α has been shown to remodel blood vessels and lymphatic vessels [19] . Its vascular remodelling function on blood vessels is mediated by TNFR1 expressed in endothelial cells, whereas remodelling of lymphatics is probably achieved by recruitment of leukocytes since LECs lack TNFR1 expression [19] . Our present findings, however, show both in vitro isolated mouse and hLECs that express TNFR1, which was further validated in several in vivo experimental models. Further, we show that TNF-α directly stimulates LEC activity, which can be inhibited by knocking down TNFR1. The discrepancy between our findings and this study is not known. However, it is highly probable that lymphatic vessels under various pathological settings possess different features and express different surface molecules. It is also possible that LECs under influence by a specific microenvironment selectively express certain signalling molecules to justify their functions. These possibilities warrant further investigation. Interestingly, two other previous studies have also implied the potential interplay between the TNF-α and the VEGF-C-VEGFR3 signalling. In a TNF-α-induced chronic arthritis genetic model, loss of function of VEGFR3 by administration of an anti-VEGFR3 neutralizing antibody significantly decreased the number of lymphatic vessels in joints [15] . However, the VEGFR3 blockade increased synovial volume and inflammation. In contrast, gain-of-function experiments by delivery of adenoviral VEGF-C increased lymphangiogenesis and lymphatic drainage, leading to attenuation of joint damage [18] . We also show that TNFR1- and VEGFR3-mediated signals are not mutually exclusive, but are mutually dependent to accomplish the TNF-α-induced lymphangiogenesis ( Fig. 8d ). Depletion of TNFR1 impairs TNF-α-induced recruitment and activation of macrophages, leading to defective production of VEGF-C and thus attenuating the VEGFR3 signalling pathway. In addition, inhibition of TNFR1 also impairs the direct effect of TNF-α on LECs. VEGFR3-mediated LEC guidance alone without TNFR1-triggered proliferative and migratory signals would be insufficient to establish a lymphatic network. Another key finding is that TNF-α markedly promotes lymphatic metastasis by inducing peri- and intratumoral lymphangiogenesis in an inflammation-dependent manner. This novel function significantly increases our understanding of the complex role of TNF-α and inflammatory macrophages in the tumour microenvironment in promoting tumour growth, invasion and metastasis. In addition to our findings, TNF-α-induced tumour cell migration and induction of CCL1 might also facilitate to lymph node metastasis [47] , [48] . Perhaps, these other mechanisms coordinate with lymphangiogenesis in promoting lymphatic metastasis. The fact that deletion of Tnfa gene in mice does not affect developmental and physiological angiogenesis and lymphangiogenesis suggests that the TNF-α-TNFR1 signalling pathway is primarily involved in pathological angiogenesis and lymphangiogenesis. In this aspect, development of drugs that target the TNF-α-TNFR1 signalling would less likely cause vasculature-related adverse effects. Our findings are clinically relevant since TNF-α-induced lymphangiogenesis was also validated in naturally occurring human ovarian tumours. Downregulation of TNF-α expression in ovarian tumours inhibited tumoral lymphangiogenesis and lymphatic metastasis. Taken together, our present data shed novel mechanistic light on understanding tumour inflammation in promoting lymphangiogenesis and complex interplay between various lymphangiogenic signals and lymphatic metastasis, and provide new conceptual information for therapeutic development of anti-metastatic drugs by targeting the TNF-α-TNFR1 signalling pathway. Cell lines Murine LLC cells transfected with BMG Neo or BMG Neo-TNF-α were kindly provided by Dr Fumiaki Koizumi at the National Cancer Center, Tokyo, Japan. LLCs were cultured in DMEM medium (Hyclone, Utah, USA) containing 20% fetal bovine serum (FBS) with 200 U ml −1 penicillin and 50 μg ml −1 streptomycin. The human telomerase-immortalized human dermal LECs (hTERT–HDLECs) were kindly provided by Dr Steen Dissing at the Panum Institute, Copenhagen University, Denmark. Primary mouse dermal LECs were isolated from the lung tissue of adult C57BL/6 healthy mice. In brief, dissected lung tissues were cut into small pieces, followed by digestion with 0.2% collagenase at 37 °C for 15–30 min. Single cell suspensions were cultured with endothelial cell growth medium 2 supplemented with 10% fetal calf serum. LYVE-1 + cells were sorted and collected by FACS [22] . hTERT–HDLECs and mouse dermal LECs were cultured onto 1% gelatine-coated dishes with a commercially available endothelial cell growth medium MV2 (Promocell, Germany). Primary HUVECs were purchased from ATCC (VA, USA); the human IGROV-1 ovarian carcinoma cell line was provided by Dr Stefano Indraccolo, Istituto Oncologico Veneto—IRCCS, Italy. Human OVCAR-8 ovarian cancer cell line was kindly provided by Dr Xuri Li at the National Institute of Health, MD, USA. IGROV-1 and OVCAR-8 ovarian cancer cell lines were cultured in RPMI medium (Hyclone) containing 10% FBS. Raw 264.7 and U937 monocytes were provided by Dr Martin Rottenberg at the Department of Microbiology, Tumor and Cell biology of Karolinska Institutet. Raw 264.7 was cultured in 10% FBS–DMEM medium and U937 was cultured in 10% FBS–RPMI medium. Cell morphology assays siRNA-transfected LEC cells were grown on coverslips in six-well plates to about 50% confluency and stimulated with 100 ng ml −1 of TNF-α (R&D systems, Minneapolis, MN, USA) or VEGF-C (PeproTech, Rocky Hill, NJ, USA). After 48 h incubation, cells were fixed with 3% paraformaldehyde (PFA) in phosphate-buffered saline (PBS, pH 7.5) for 30 min at room temperature. After rinsing three times with PBS, the cells were permeabilized with 0.5% Triton X-100 for 30 min. Cells were stained for 30 min with 1 μg ml −1 of rhodamine-phalloidin (Sigma, Santa Clara, CA, USA) in PBS. After rigorous washing, randomized representative fields were photographed using a fluorescent microscope (Nikon D-eclipse C1, Tokyo, Japan). Percentages of cells with elongated morphologies were calculated from total cell numbers from six randomized fields of three independent samples per group. Immunostaining of cells in vitro HUVECs, hLECs and U937 cells grown in monolayers on coverslips were fixed with 3% PFA for 30 min, followed by washing with PBS for three times. For staining with an anti-Prox-1 antibody (rabbit anti-mouse Prox-1 antibody, Abcam, Cambridge, MA, USA; 1:200), LECs were fixed with 100% methanol for 30 min. The methanol-fixed cells were blocked with 4% goat serum for 30 min. PFA-fixed cells were blocked with 1% skim milk in PBS and stained with a goat anti-human TNFR1 antibody (R&D systems; 1:200) or a goat anti-human TNFR2 antibody (R&D systems; 1:200). Stained cells were rinsed with PBS for several times and incubated with a second antibody of donkey anti-goat Alexa Fluor 555-conjugated antibody (Invitrogen, Carlsbad, CA, USA; 1:400). After rigorous washing, cells were analysed under a fluorescent microscope (Nikon D-eclipse C1). Randomized representative fields were photographed. Migration assay LEC migration assay was performed by a modified Boyden chamber technique [22] , [44] . LEC at the density of ~3 × 10 4 cell together with 100 ng of TNF-α (R&D systems) or VEGF-C (PeproTech) with or without various antibody blockades at the concentration of 1 μg ml −1 was added to each upper chamber. After 4 h incubation, the Boyden chamber was disassembled and migrated cells were stained with Giemsa (Sigma) and counted under a light microscope (Nikon eclipse TS100). For quantification analysis, at least six independent samples per group were used. The same migration protocol was also used to study Raw 264.7 migration in response to various stimuli. Cell proliferation assay Cell proliferation assay was performed with the MTT (3-(4,5-dimethylthiazol-2-yl)-2,5-diphenyltetrazolium bromide) method [22] . Briefly, MTT (Sigma) was used for human and mLEC proliferation assay. Approximately 3,000 LECs were seeded onto each well of gelatine-coated 96-well plates in a total volume of 200 μl Endothelial Cell Growth Medium (PromoCell) containing 2% fetal calf serum for 1 day. Cells were treated with 100 ng ml −1 recombinant TNF-α (R&D systems) or VEGF-C (PeproTech) in the presence or absence of 1 μg ml −1 rat anti-mouse neutralizing VEGFR3 antibody (Imclone, NY, USA). Cells were counted at 72 h post incubation. For Coulter counter method [49] , tumour cell proliferation was assayed at 72 h after incubation. In brief, transfected and non-transfected tumour cells were seeded at a density of 1 × 10 4 cells per well in 24-well plates in DMEM medium (10% FBS), and incubated at 37 °C. Cells were trypsinized, resuspended in Isoton II solution (Beckman Coulter, Sweden) and counted in a Coulter counter at the indicated time points. Triplicates were used for each sample. Enzyme-linked immunosorbent assay Tumour tissue or sorted cells were collected for enzyme-linked immunosorbent assay (ELISA) using ELISA kit for analysis of human TNF-α (R&D Systems) or mouse VEGF-C (Mybiosource, CA, USA) according to the instructions from the manufacturer. For tumour tissue ELISA, ~50 mg of the non-necrotic fresh tumour tissue was homogenized in 500 μl lysis buffer (CelLytic MT mammalian tissue lysis/extraction reagents, Sigma) in the presence of a cocktail of proteinase inhibitors (Sigma). For sorted cells’ ELISA, F4/80 + cells were sorted from ~1 g of tumour tissue. Cells were count and homogenized in 100 μl lysis buffer. Samples were homogenized, then centrifuged at 12,000 r.p.m. for 15 min. Supernatants were used for ELISA analysis as mentioned above. Animals All animal studies were approved by the North Stockholm Animal Ethical Committee. C57BL/6 mice were provided by the breeding unit of the animal facility of Department of Microbiology, Tumor and Cell Biology, Karolinska Institute, Sweden; B6.129S2- Tnfrsf1b tm1Mwm /J ( Tnfr1 −/− ) mice in C57BL/6 background were purchased from the Jackson Laboratory (Bar Harbor, Maine, CA, USA); and immunodeficient CB17/Icr-Prkdcscid/IcrCrl mice were obtained from Charles River Laboratories. Female mice at age 6–8 weeks were used for all tumour studies. Male C57BL/6 mice at age 6–8 weeks were used for corneal studies. Mouse corneal micropocket assay The mouse corneal micropocket assay was performed by implanting micropellets into mouse cornea [22] , [25] , [50] . In brief, a slow-release polymer-made micropellet containing 40 ng of TNF-α (R&D systems) or 160 ng of VEGF-C (PeproTech) was implanted into each corneal micropocket, which was surgically created on a single eye of each animal ( n =4 mice per group). Corneal neovascularization was measured on day 6 after pellet implantation. Subgroups of implanted animals were systemically treated with an anti-VEGFR3 neutralizing antibody (300 μg per mouse) by intraperitoneal injection on postoperative days 0, 2 and 4 (ref. 32 ). Mouse tumour experiments C57BL/6 or severe combined immunodeficiency mice at age 6–8 weeks were subcutaneously injected with 1 × 10 6 vector-, TNF-α or VEGF-C-stably expressing tumour cells into the dorsal middle region of each mouse. Tumour growth rates were measured every other day and tumour volumes were calculated according to the standard formula tumour volume=length × width 2 × 0.52 (ref. 51 ). Tumour vascular perfusion was measured by injecting 2,000 kD lysine-fixable tetramethylrhodamine-dextran (Invitrogen) and vascular permeability was measured by extravasation of 70 kD lysinated dextran. Briefly, 100 μl of 2,000 kD dextran was injected into the tail vein of each mouse 5 min before they were killed. For 70 kD dextran, injection was performed 15 min before they were killed. Tumour tissues were immediately fixed with 4% PFA (wt/vol) at 4 °C overnight and further assessed by whole-mount analysis. For measurement of lymphatic drainage, each tumour implanted in the ear received injection of 50 μl of Indian ink [29] . The mice were placed in a warm pad and lymphatic drainage was measured 5 min after injection with Indian ink by taking pictures. Dye-drained lymphatic vessels were easily detectable and counted (eight mice per group). Tumour interstitial fluid pressure (IFP) was measured with a needle-probe pressure monitor system (Evolution Chassis, FISO Technologies, QC, Canada). Tumour-bearing mice were anaesthetized with isoflurane and the needle probe was inserted into the centre of each tumour. IFP was recorded when the measurement stabilized. Metastasis Tumour-bearing mice were anaesthetized with hypnorm-dormicum (Vetapharma, Leeds, UK) at 1:1 ratio. Primary tumours at the volumes of 1.0–1.5 cm 3 were surgically removed under this anaesthetic condition and mice received an additional pain killer (Temgesic (Reckitt Benckiser, Berkshire, UK), 0.1 mg kg −1 , twice a day) in 2 consecutive days after operation. Approximately 3–4 weeks after tumour removal, visible metastases could be detected in some axillary lymph nodes of a subpopulation of TNF-α tumour-bearing mice or other tumour-bearing mice. Mice were killed at this time and axillary lymph nodes as well as other organs including lung, liver, spleen, kidney and brain were dissected and analysed for EGFP + tumour metastases under a fluorescent microscope and histological examination. In all experiments, 6–12 mice were used in each group. Drug treatments Clodronate liposome (dichloromethylene bisphosphonate; ClodronateLiposomes, the Netherlands) solution at the concentration of 6 mg ml −1 clodronate liposomes was used to treat the mice. Clodronate liposomes or control PBS liposomes in 100 μl were intravenously injected through tail vein into each mouse that had received the same volume of clodronate liposomes the day before by subcutaneous injection to deplete local macrophages. Clodronate liposome intravenous injections continued once every 5–7 days in tumour-bearing mice starting from the day before tumour cell implantation. A rat anti-mouse VEGFR3 neutralizing antibody (mF4-31C1; ImClone) was intraperitoneally injected at a dose of 300 μg per mouse [22] . Monocyte/macrophage transplantation Whole blood was collected by intracardiac puncturing using heparinized syringes from wt or Tnfr1 −/− mice. Monocyte/macrophage/eosinophil populations were stained with an anti-F4/80 (Biolegend, San Diego, CA, USA) antibody, followed by FACS. Approximately 1 × 10 5 of isolated F4/80 + cells were intravenously injected into the Tnfr1 −/− mice once per week for 4 weeks. TNF-α-expressing tumour cells at the density of 1 × 10 6 in 100 μl PBS were subcutaneously implanted into each mouse the day after the first monocyte/macrophage injection. When tumour reached to 1 cm 3 , tumour-bearing mice were killed and tumours were removed. Fresh tumour tissues were whole-mount stained with different antibodies. Histology and whole-mount staining Histology and whole-mount immunostaining were performed according to our standard protocol [25] , [52] , [53] . In brief, paraffin-embedded tissues were sectioned at the thickness of 4 μm and stained with hematoxylin and eosin stain. Freshly prepared tumour, lymph node and corneal tissues were sliced into small pieces and whole-mount stained with CD31, LYVE-1, F4/80, VEGFR3 and CD206. A rat anti-mouse CD31 monoclonal antibody (BD Pharmingen, Franklin Lakes, NJ, USA; 1:200), a hamster anti-mouse CD31 antibody (Millipore, Billerica, MA, USA; 1:200), a rabbit anti-mouse LYVE-1 antibody (AngioBio, Del Mar, CA, USA; 1:100), a goat anti-human TNFR1 antibody (R&D systems; 1:200), a goat anti-human TNFR2 antibody (R&D systems; 1:200), a goat anti-mouse TNFR1 antibody (R&D systems; 1:200), a goat anti-mouse TNFR2 antibody (R&D systems; 1:200), a goat anti-mouse VEGFR3 antibody (R&D systems; 1:200), a rat anti-mouse F4/80 antibody (AbD serotec, Oxford, UK; 1:200), a rabbit anti-mouse F4/80 antibody (Novus Biologicals, Littelton, CO, USA; 1:200), a rat anti-mouse CD206 antibody (Biolegend; 1:200) and a rat anti-mouse Ki67 antibody (eBioscience, San Diego, CA, USA; 1:200) were used as primary antibodies. A goat anti-rat Alexa Fluor 555-conjugated antibody (Invitrogen; 1:400), a goat anti-rabbit Alexa Fluor 488-conjugated antibody (Invitrogen; 1:400), a Cy3-conjugated goat anti-rabbit IgG antibody (Chemicon, Temecula, CA, USA; 1:400), a Cy3-conjugated goat anti-hamster antibody (Jackson ImmunoResearch, West Grove, PA, USA; 1:200), a donkey anti-goat Alexa Fluor 555-conjugated antibody (Invitrogen; 1:400), a donkey anti-rabbit Alexa Fluor 488-conjugated antibody (Invitrogen; 1:400), a donkey anti-rat Alexa Fluor 647-conjugated antibody (Invitrogen; 1:400), a donkey anti-rat Alexa Fluor 555-conjugated antibody (Invitrogen; 1:400) were used as secondary antibodies. Stained tissue samples were examined under a confocal microscope (Nikon D-eclipse C1), using Confocal software (EZ-C1 3.9 Nikon digital eclipse). Real-time qPCR and RT–PCR Real-time qPCR and RT–PCR were performed according to the standard protocols with commercially available kits [54] . Sample RNA preparation was performed by a GeneJet RNA Purification Kit (Thermo Scientific, MA, USA), and complementary DNA synthesis was achieved by a RevertAid H minus First Strand cDNA Synthesis Kit (Thermo Scientific, MA, USA). PCR was performed using a DreamTaq Green PCR Master Mix Kit (Thermo Scientific, MA, USA) and 2720 PCR machine (Applied Biosystems, CA, USA), qPCR was performed by a Power SYBR Green Master Mix Kit (Applied Biosystems) and a Step One Plus real-time PCR system (Applied Biosystems) [54] . The primer pairs specific for various genes used in our experiments are shown in Supplementary Table 1 . A triplicate sample was analysed in each group. siRNA and shRNA interference siRNA targeting human TNFR1, TNFR2, VEGFR3, scrambled siRNA and transfecting medium were purchased from Dharmacon (Thermo Scientific, Lafayette, CO, USA) and transfection was performed according to the manufacturer’s instructions [54] , [55] . For shRNA experiments, plasmids containing shRNA specific for human TNFα and a lentiviral vector-based expression packaging kit were purchased from GeneCopoeia (catalogue no. HSH018141, Rockville, MD, USA). Experiments were performed according to the manufacturer’s instructions [54] . Detection of activated PLCγ1 in LECs Human dermal LECs (hLECs) were treated with 100 ng ml −1 TNF-α (R&D systems) for 0, 15 or 30 min. Total protein lysates were subjected to SDS–polyacrylamide gel electrophoresis (Invitrogen) with subsequent transfer onto nitrocellulose membranes (PerkinElmer, Waltham, MA, USA). Blocking was performed with 5% bovine serum albumin (Sigma) for 30 min at room temperature followed by incubation with specific primary antibodies for detection of total PLC γ1 (Millipore, Billerica, Massachusetts, USA; 1 μg ml −1 ), P-PLC γ1 (Millipore; 0.5 μg ml −1 ) or β-actin (Cell Signaling, Cambridge, UK; 1:1,000) over night at 4 °C. Membranes were incubated with an anti-mouse secondary antibody conjugated to IRDye 680RD (LI-COR, Lincoln, NE, USA; 1:15,000) and visualized and quantified using Odyssey CLx detection system (LI-COR, Lincoln). Pull down and detection of GTP-Rac1 About 1 × 10 6 hLECs were treated with 100 ng ml −1 TNFα for 0 or 2 min. Subsequent extraction and affinity purification were performed according to the manufacturer’s instructions using a Rac1/Cdc42 Activation Assay Kit (Millipore). In brief, cellular proteins were extracted with a Mg 2+ Lysis/Wash Buffer (MLB) and pre-cleared with glutathione agarose (Sigma). Total lysates were saved for protein concentration measurements and detection of total Cdc42/Rac1. Affinity purification of activated Cdc42/Rac1 in aliquots of cell extracts was performed by addition of PAK-1 PBD agarose with incubation at 4 °C. Beads were resuspended in reducing sample buffer. Total and affinity-purified samples were subjected to SDS–polyacrylamide gel electrophoresis as described above. Anti-Cdc42 (Millipore; 1 μg ml −1 ) and anti-Rac1 (Millipore; 1 μg ml −1 ) were incubated overnight at 4 °C, followed by incubation with a rhodamine-conjugated anti-mouse secondary antibody IRDye 680RD (LI-COR, Lincoln; 1:15,000). Positive signals were detected with Odyssey CLx system (LI-COR, Lincoln). All original pictures of immunoblots are shown in Supplementary Fig. 9 . FACS analysis and FACS Mice ( n =6 per group) were killed by CO 2 overdose at the end of the experimentation. For analysis of tumour tissue cells including TAMs, single cell suspensions were prepared by 0.15% collagenase I and II digestion of small pieces of tumour tissue at 37 °C for 60 min, and followed by filtration with a 40-μm diameter cell filter [53] . Single cell suspensions were subjected to FACS analysis according to our previous published methods using FACSort and CellQuest software (BD Bioscience, Franklin Lakes, NJ, USA). For isolation of F4/80 + cells from peripheral blood, whole blood was collected by heart puncture using heparinized syringes. Single cell suspensions were prepared by red blood cell (RBC) lysis buffer. About 2.5 ml of RBC lysis buffer was added to 250 μl blood sample. The lysis process was stopped after 2–5 min incubation at room temperature by adding 10 ml PBS, followed by centrifugation at 1,500 r.p.m. for 5 min. Cell pellets were resuspended in PBS [53] . For isolation of TAMs, single cell suspensions were prepared by above mentioned collagenase digestion method. After FACS, cells were centrifuged and the platelet is immediately used for further analysis. An anti-mouse Alexa Fluor 647-conjugated F4/80 antibody (Biolegend; 0.25 μl for 1 × 10 6 cells) and an anti-mouse Alexa Fluor 488-conjugated CD206 antibody (Biolegend; 1 μl for 1 × 10 6 cells) were used in the FACS analysis and FACS. Statistical analysis Quantification analyses were performed as follows: six randomized fields of three independent samples per group for in vitro LEC morphology; four independent mice per group for quantification of corneal angiogenesis and lymphangiogenesis; eight randomized micrograph fields from 6–8 different tumour samples for whole mount; 12–24 lymph nodes (6–12 mice; 2 subaxillary lymph nodes per mouse). The Adobe Photoshop CS4 software program was used with a colour range tool and a count tool to detect positive areas or numbers. Statistical differences between two groups were assessed by unpaired Student’s t -test, and comparison of multiple groups involved the use of analysis of variance and values of * P ≤0.05, ** P ≤0.01 and *** P ≤0.001 were deemed statistically significant. How to cite this article : Ji, H. et al. TNFR1 mediates TNF-α-induced tumour lymphangiogenesis and metastasis by modulating VEGF-C-VEGFR3 signalling. Nat. Commun. 5:4944 doi: 10.1038/ncomms5944 (2014).